RhoGAP domain-containing fusions andPPAPDC1Afusions are recurrent and prognostic in diffuse gastric cancer We conducted an RNA sequencing study to identify novel gene fusions in 80 discovery dataset tumors collected from young patients with diffuse gastric cancer (DGC). Twenty-five in-frame fusions are associated with DGC, three of which ( CLDN18-ARHGAP26, CTNND1-ARHGAP26 , and ANXA2-MYO9A ) are recurrent in 384 DGCs based on RT-PCR. All three fusions contain a RhoGAP domain in their 3’ partner genes. Patients with one of these three fusions have a significantly worse prognosis than those without. Ectopic expression of CLDN18-ARHGAP26 promotes the migration and invasion capacities of DGC cells. Parallel targeted RNA sequencing analysis additionally identifies TACC2-PPAPDC1A as a recurrent and poor prognostic in-frame fusion. Overall, PPAPDC1A fusions and in-frame fusions containing a RhoGAP domain clearly define the aggressive subset (7.5%) of DGCs, and their prognostic impact is greater than, and independent of, chromosomal instability and CDH1 mutations. Our study may provide novel genomic insights guiding future strategies for managing DGCs. Gastric cancer presents in two major histological subtypes, intestinal and diffuse-type gastric cancers (DGCs). Despite the relatively high incidence of DGC [1] , [2] , few whole transcriptomic analyses have been performed for this histological subtype. We therefore conducted an RNA sequencing study to search for novel driver fusions in DGC. Several fusions have previously been reported to drive gastric cancer [3] , [4] , [5] , [6] , [7] , [8] , but few of these have been validated by subsequent studies [3] , [9] . The Cancer Genome Atlas (TCGA) Research Network discovered that a cryptic splice site within exon 5 of CLDN18 activates the ARHGAP26 or ARHGAP6 splice acceptor, leading to the expression of CLDN18-ARHGAP fusion transcripts in gastric cancer, especially in the genomically stable (GS) tumors [3] . The CLDN18-ARHGAP fusions retain the transmembrane domains of CLDN18 and the Rho GTPase activating protein (RhoGAP) domain of ARHGAP26/6 [3] . Yun et al. found the PPP1R1B-STARD3 read-through fusion in 21.3% of gastric cancer tissues [5] . Palanisamy et al. reported that a gastric cancer expresses the AGTRAP-BRAF fusion containing the C-terminal kinase domain of BRAF (7q34) fused to the N-terminal angiotensin II type 1 receptor-associated domain of AGTRAP (1p36) [6] . The CD44-SLC1A2 fusion, which results from 11p13–15 chromosomal inversion, is found in 1–2% of gastric cancer [7] . The SLC34A2 (4p15)- ROS1 (6q22) fusion is present in 0.4% of gastric cancer and is associated with ROS1 protein overexpression [8] . Except for the CLDN18-ARHGAP fusions [9] , these in-frame gene fusions have not been validated by subsequent gastric cancer publications. Younger cancer patients express certain gene fusions at a higher frequency than older patients, including ALK or RET fusions in lung adenocarcinomas [10] , [11] , RET/PTC1 and RET/PTC3 fusions in papillary thyroid cancer [12] , EWSR1/FUS-ATF1 fusions in mesothelioma [13] , and DUX4 fusions in B cell acute lymphoblastic leukemia [14] . Despite a trend for the prevalence of gene fusions in young cancer patients, no studies have systematically investigated novel fusions in young patients with DGCs due to the relative rarity of early-onset gastric cancer, which is notable for its strong enrichment of diffuse histology. We previously published a whole exome sequencing study demonstrating that CDH1 mutations are highly prevalent in early-onset DGCs [15] . CDH1 and RHOA mutations underlie unique phenotypes of DGC, such as poorly cohesive growth, but there is a subset of DGCs that are wild-type for CDH1 and RHOA [15] . RNA sequencing of an early-onset DGC discovery set To identify somatic alterations in transcriptomic profiles in early-onset DGC, we performed RNA sequencing on DGCs collected from 80 young ( ≤ 45 years) Korean patients who had not been treated with chemotherapy or radiation [15] . The median age of this population was 38 years (range, 20‒45) and 58.7% was female, as previously reported [15] . When the sequencing data were aligned using the Burrows-Wheel Aligner (BWA) to the human reference genome, hg19, median coverage of exons was 104 × [interquartile range, 91–132] and the median number of genes with ≥ 10 × coverage was 15,960 [interquartile range, 15,401–16,600]. The median total exon coverage and 5’/3’ coverage ratio were 91% [interquartile range, 90%–92%] and 0.75 [interquartile range, 0.68–0.82], respectively. Microsatellite unstable tumors (MSI) have a strong immune gene expression signature and favorably respond to anti-PD-1 therapy, but the MSI tumors are relatively rare in DGC, especially in early-onset DGC [15] . Hierarchical clustering analyses of the Reads Per Kilobase Million (RPKM) data of our discovery dataset revealed four distinct clusters. One key cluster characterized by overexpression of immune-related genes included all MSI (n = 2) and Epstein-Barr virus (EBV)-positive tumors (n = 7; Supplementary Fig. 1 and Supplementary Tables 3 and 4 ). Thus, a distinct cluster expressing a strong immune gene signature existed even in early-onset DGCs. We also performed RNA sequencing on 65 samples of normal tissue adjacent to the 80 tumors that had RNA sequencing data. We applied bioinformatics algorithms such as PRADA and Trans-ABySS to the RNA-sequencing dataset to predict novel in-frame fusions, and performed RT-PCR to validate the expression of these in-frame fusion candidates (Supplementary Table 5 ). 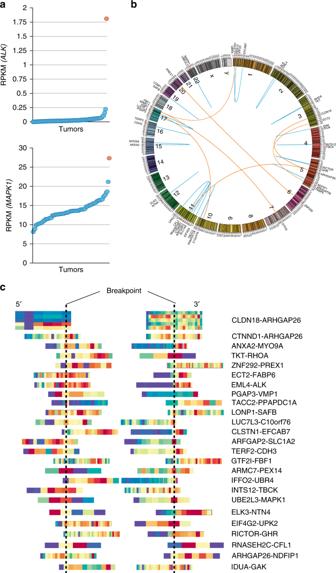Fig. 1 Twenty-five in-frame gene fusions identified in a discovery dataset of 80 early-onset DGCs (a) Top panel, Expression level ofALKin the tumor containing theEML4-ALKfusion (magenta circle). Each circle represents each tumor. Sample ordering according toALKexpression level. Bottom panel, Expression level ofMAPK1in the tumor containing theUBE2L3-MAPK1fusion (magenta circle). Sample ordering according toMAPK1expression level. (b) Circos plot for the 25 in-frame fusions. (c) Exon-level, Fragments Per Kilobase Of Exon Per Million Fragments Mapped (FPKM) values for the in-frame gene fusions. Heatmap after gene centering. Dotted lines, mRNA breakpoints; Red, higher expression level; Blue, lower expression level. In a majority of fusions, 3’ partner genes overexpressed exons that were located 3’ to the breakpoints Twenty-five in-frame fusions were confirmed in 20 tumors from our early-onset DGC population (Table 1 ). Twenty-four of these in-frame fusions were novel to gastric cancer. 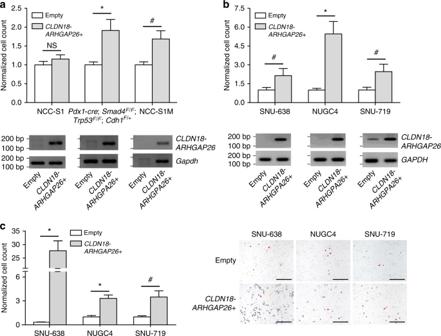Fig. 5 Functional effects ofCLDN18-ARHGAP26overexpression (a) Top, Trans-well migration assay. Mouse gastric cancer cells stably expressingCLDN18-ARHGAP26demonstrated significantly enhanced migration ability compared with those expressing an empty vector (P < 0.001, Wilcoxon signed rank), and this effect was prominent in NCC-S1M andPdx1-cre;Smad4F/F;Trp53F/F;Cdh1F/+cells. Vertical axis denotes the normalized number of migrated cells per field. Average values of 4 independent experiments; Bottom, RT-PCR forCLDN18-ARHGAP26(b) Top, Migration assay of human gastric cancer cells following the ectopic expression ofCLDN18-ARHGAP26. Human gastric cancer cells stablyCLDN18-ARHGAP26demonstrated significantly enhanced migration capacity compared with those expressing an empty vector (P < 0.001, Wilcoxon signed rank). Vertical axis denotes the normalized number of migrated cells per field. Average values of 3 independent experiments; Bottom, RT-PCR forCLDN18-ARHGAP26. (c) Left, Invasion assay. Human gastric cancer cells stably expressingCLDN18-ARHGAP26demonstrated significantly enhanced invasion capacity compared with those expressing an empty vector (P < 0.001, Wilcoxon signed rank). Vertical axis denotes the normalized number of migrated cells per field. Average values of three independent experiments. Right, Representative photographs of the invasion assay (200 × , scale bar = 0.2 mm). Red arrows, gastric cancer cells. Error bars, mean ± SEM.#P < 0.05, *P < 0.01, **P < 0.001, ***P < 0.0001 Only the CLDN18-ARHGAP26 fusion had previously been associated with gastric cancer by The Cancer Genome Atlas (TCGA) project [3] . Notably, one of the novel in-frame fusions, EML4-ALK , was clinically-actionable but had not been previously associated with gastric cancer [16] . A tumor containing the EML4-ALK fusion had the highest ALK expression (Fig. 1a ). Table 1 In-frame fusions in a discovery set (n = 80) Full size table Fig. 1 Twenty-five in-frame gene fusions identified in a discovery dataset of 80 early-onset DGCs ( a ) Top panel, Expression level of ALK in the tumor containing the EML4-ALK fusion (magenta circle). Each circle represents each tumor. Sample ordering according to ALK expression level. Bottom panel, Expression level of MAPK1 in the tumor containing the UBE2L3-MAPK1 fusion (magenta circle). Sample ordering according to MAPK1 expression level. ( b ) Circos plot for the 25 in-frame fusions. ( c ) Exon-level, Fragments Per Kilobase Of Exon Per Million Fragments Mapped (FPKM) values for the in-frame gene fusions. Heatmap after gene centering. Dotted lines, mRNA breakpoints; Red, higher expression level; Blue, lower expression level. In a majority of fusions, 3’ partner genes overexpressed exons that were located 3’ to the breakpoints Full size image Of the novel in-frame fusions listed in Table 1 , the following had not been previously identified in any tumor type: CTNND1-ARHGAP26, TKT-RHOA, ARFGAP2-SLC1A2 [7] , IFFO2-UBR4 [17] , PGAP3-VMP1 [17] , UBE2L3 [18] - MAPK1, ZNF292-PREX1 [19] , TACC2-PPAPDC1A [20] , ANXA2-MYO9A , ECT2-FABP6 , LONP1-SAFB , LUC7L3-C10orf76 , CLSTN1-EFCAB7 , TERF2-CDH3 , GTF2I-FBF1 , ARMC7-PEX14 , INTS12-TBCK , ELK3-NTN4, EIF4G2-UPK2, RICTOR-GHR, RNASEH2C-CFL1, ARHGAP26-NDFIP1 , and IDUA-GAK (Fig. 1b ). The first eight fusions, which had ARHGAP26, RHOA, SLC1A2, UBR4, PGAP3, UBE2L3, PREX1 and PPAPDC1A as fusion partners, were previously reported with different fusion partners by the gastric cancer TCGA project ( CLDN18-ARHGAP26, PRKAR2A-RHOA, CD44-SLC1A2, PIK3CD-UBR4, STARD3-PGAP3 , and HNF1B-PGAP3 ) or in the literature [7] , [17] , [18] , [19] , [20] , [21] . These findings suggest that the dysregulation of the identified genes may have functional roles in gastric cancer. Most of these 25 in-frame fusions overexpressed their 3’ partner genes (Fig. 1c ). As with EML4-ALK , the UBE2L3 - MAPK1 fusion-containing DGC expressed the highest level of MAPK1 within the discovery set (Fig. 1a ). 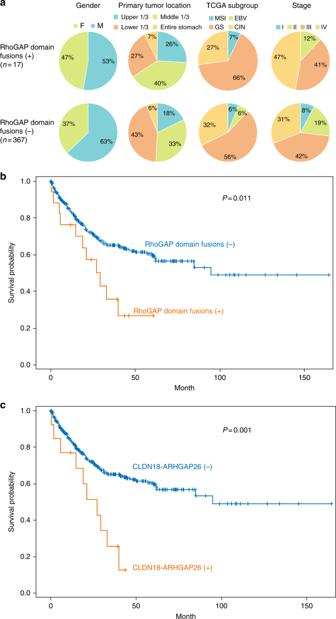Similarly, the ARFGAP2-SLC1A2 fusion-containing DGC expressed the second highest level of SLC1A2 (Supplementary Fig. Fig. 4 Clinical implications of RhoGAP domain-containing fusions in the expanded dataset (n = 384) (a) Clinicopathological characteristics (gender and primary tumor location) and TCGA subgroups in patients with (upper row) and without (lower row) RhoGAP domain-containing fusions. (b) Kaplan-Meier curves for the overall survival of patients with DGCs expressing three recurrent RhoGAP domain-containing fusions (n = 17) and those without (n = 367). (c) Kaplan-Meier curves for the overall survival of patients with DGCs expressing theCLDN18-ARHGAP26fusion (n = 13) and those without (n = 371) 2 ). Notably, several studies have reported SLC1A2 , a glutamate transporter, as a common 3’ partner gene for fusions in solid tumors. For example, CD44-SLC1A2 fusion is found in both gastric [7] and colorectal cancers [22] . Thus, SLC1A2 fusions may drive DGC carcinogenesis. Interestingly, other previously reported clinically-actionable fusions were not present in our discovery set. Fusions involving BRAF and ROS1 have been reported in gastric cancers [6] , [8] , but were not observed in any of the 80 DGCs we analyzed. DAVID gene ontology analysis revealed that many 3’ partner genes of these 25 fusions were significantly enriched within the Rho GTPase pathway (P = 0.01, Supplementary Table 6 ). Specifically, ARHGAP26, RHOA, PREX1, MYO9A, ECT2 , and CFL1 were Rho GTPases or their regulators and downstream effectors. 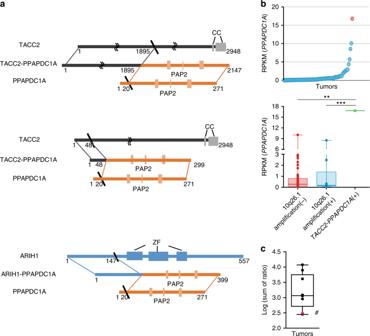Fig. 6 ThePPAPDC1Ain-frame fusions identified by targeted RNA sequencing (a) Schematic representation of thePPAPDC1Afusions. Top and middle panels,TACC2-PPAPDC1Afusions; Bottom panel,ARIH1-PPAPDC1A. CC, Coiled-coil domain; PAP2, PAP2 domain; ZF, Zinc finger domain. (b) Left,PPAPDC1ARPKM values for the 80 discovery set DGCs. Each circle represents each tumor. Sample ordering according to thePPAPDC1ARPKM. Magenta circle, early-onset DGC expressingTACC2- PPAPDC1A. Right,PPAPDC1ARPKM values for the discovery set DGCs with and without 10q26.1 gene amplification. Turquoise circle, early-onset DGC expressingTACC2- PPAPDC1A. Box plots display 5%, 25%, median, 75%, and 95%. (c) Lipidomic profiling data for DGCs with or withoutTACC2-PPAPDC1A. The sum of the mass spectral peak area ratio between phosphatidic acid (PA, the substrate of PPAPDC1A) and diacylglycerol (DG, the product of PPAPDC1A) was significantly lower in an early-onset DGC expressingTACC2-PPAPDC1Ain the discovery set than in randomly-selected eight DGCs without the fusion (P = 0.01, one-sample rank sum test). Vertical axis denotes the sum of mass spectral peak area ratio between PA and the corresponding DG for each PA-DG pair. Each circle represents each tumor. Magenta circle, early-onset DGC expressingTACC2- PPAPDC1A.#P value for an one-sample rank sum test. Box plots display 5%, 25%, median, 75%, and 95% These results suggest that the Rho GTPase pathway is altered by gene fusion events in a subset of DGCs. Recurrent in-frame fusions in DGC To evaluate the clinical and biological implications of these fusions in a larger sample set of DGCs, we expanded our dataset to include 384 Korean patients. Whereas this expanded dataset included all 80 early-onset DGCs in a discovery dataset, the expanded dataset comprised predominantly (n = 249) of older patients ( ≥ 46 years of age) with late-onset DGC. We performed RT-PCR on these 384 tumors to analyze the expression of the in-frame fusions previously identified in our early-onset DGCs (Supplementary Table 1 ). Three of these fusions, CLDN18-ARHGAP26, CTNND1-ARHGAP26 , and ANXA2-MYO9A , were recurrent ( i.e ., present in ≥ 2 samples) in this expanded dataset (Fig. 2 and Supplementary Fig. 3 ). Of the 384 DGCs, 17 tumors (4.4%) harbored one of these three in-frame fusions. None of these three fusions were identified in adjacent normal tissue from the corresponding 17 tumors, suggesting that these fusions represent somatic alterations. Fig. 2 Schematic representation of three recurrent RhoGAP domain-containing fusions ( a ) Chromatogram for the RT-PCR sequencing data. Dotted red lines, mRNA breakpoints. ( b ) Top panel, the CLDN18-ARHGAP26 fusion. Middle panel, the CTNND1-ARHGAP26 fusion was composed of the Armadillo (Arm) family domain of CTNND1 that is involved in cell-cell adhesion and signal transduction and RhoGAP and SH3 domains of ARHGAP26 . Bottom panel, the ANXA2-MYO9A fusion was composed of 99 amino acids in the N-terminal portion of ANXA2 and the protein kinase C conserved region 1 (C1) and RhoGAP domain of MYO9A . ( c ) Left panel, Age at the time of diagnosis was significantly lower in patients with the CLDN18-ARHGAP26 fusion (n = 13; left) than in those without (n = 371; right) (P = 0.042, Wilcoxon). Right panel, Age tended to be lower in patients with RhoGAP domain-containing fusions (n = 17; left) than those without (n = 367; right) (P = 0.10, Wilcoxon). Box plots display 5%, 25%, median, 75%, and 95%. (d) RhoTekin assay in 293FT cells following the ectopic expression of Anxa2-Myo9a fusion. Relative value of GTP-RHOA to total RHOA as measured by a densitometry in three independent experiments. Error bars, mean ± SEM. ( e ) RPKM values for MYO9A in 80 early-onset DGCs (dots) in a discovery dataset. Each circle represents each tumor. Blue circle, a tumor expressing the ANXA2-MYO9A fusion. ( f ) PCR sequencing chromatogram for genomic DNA isolated from a tumor expressing the ANXA2-MYO9A fusion. Dotted line, chromosomal breakpoint. ( g ) MYO9A immunohistochemistry images were taken at 200 × . Left, Two DGCs expressing the ANXA2-MYO9A fusion. Right, Representative photographs for a randomly-selected DGC without the ANXA2-MYO9A fusion (P = 0.013; ANXA2-MYO9A -positive tumors vs. ANXA2-MYO9A -negative tumors; Cochran-Mantel-Haenszel). # P < 0.05, *P < 0.01, **P < 0.001, ***P < 0.0001, Error bar, mean ± SEM Full size image The most common fusion, CLDN18-ARHGAP26 , was significantly more prevalent in early-onset DGC (8 of 135) than late-onset DGC (5 of 249; P = 0.042, chi-square). Of the 13 patients with tumors expressing a CLDN18-ARHGAP26 fusion, median patient age (38 years) was significantly lower than for the 371 patients without this fusion (54 years; P = 0.042, Wilcoxon; Fig. 2c ). Interestingly, CLDN18-ARHGAP26 was more prevalent among tumors with H. pylori than those without (P = 0.034, Fisher’s exact test; Supplementary Table 7 ). Functional studies demonstrate that the ectopic expression of CLDN18-ARHGAP26 modestly but significantly impaired the aggregation of mouse DGC cell lines (P < 0.001, t- test; Fig. 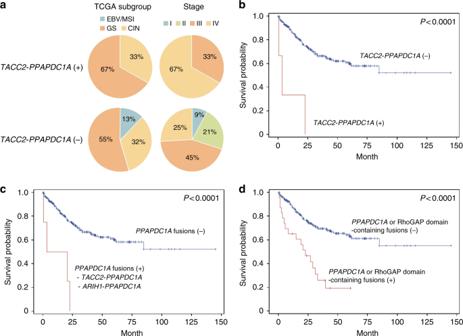Fig. 7 Clinical implications of theTACC2-PPAPDC1Afusion in the sequenced dataset (n = 305) (a) Stage at the time of diagnosis and TCGA subgroups in patients with or withoutTACC2-PPAPDC1A. TCGA subgroup was determined only in DGCs with available SNP6.0 data. (b) Kaplan-Meier curves for the overall survival of three patients with DGCs expressingTACC2-PPAPDC1Aand those without (n = 302). Their median survival times were 3.5 months and not reached, respectively (P < 0.0001, log-rank). (c) Kaplan-Meier curves for the overall survival of four patients with DGCs expressingPPAPDC1Afusions and those without (n = 301). Their median survival times were 12.1 months and not reached, respectively (P < 0.0001, log-rank; HR, 6.6 [95% CI, 2.4‒18.1]). (d) Kaplan-Meier curves for the overall survival of 23 patients with thePPAPDC1Aor RhoGAP domain-containing fusions and those without (n = 282). Their median survival times were 22.8 months [95% CI, 5.7‒33.0] and not reached, respectively (P < 0.0001, log-rank; HR, 3.4 [95% CI, 2.0‒5.7]) 3a and Supplementary Fig. 6 ), particularly in two cell lines ( Pdx1-cre; Smad4 F/F ; Trp53 F/F ; Cdh1 F/+ cells and NCC-S1 cells). Given that poorly cohesive cell growth is characteristic of DGC, these findings collectively suggest that relatively high prevalence of the CLDN18-ARHGAP26 fusion in young DGC patients underlies the strong enrichment of diffuse histology observed in early-onset gastric cancer. By contrast, the ectopic expression of CLDN18-ARHGAP26 did not enhance the tumorigenic potential of DGC cells (Supplementary Table 8 ). ARHGAP26 was also fused to another 5′ partner gene, CTNND1 , that is located at chromosome 11. The mRNA breakpoint position in ARHGAP26 (g.chr 5:142,393,645) was the same location for both CTNND1-ARHGAP26 and CLDN18-ARHGAP26 fusions. Whole genome sequencing (WGS) analysis of a tumor expressing the CTNND1-ARHGAP26 fusion revealed that g.chr11:57,578,103 ( CTNND1 intron 15) was aberrantly fused to g.chr5:142,358,707 ( ARHGAP26 intron 11; Supplementary Table 9 ) at the genomic DNA level. The CTNND1-ARHGAP26 fusion was expressed in 2 of 384 DGCs. Thus, ARHGAP26 was involved in two distinct interchromosomal translocation events in our expanded DGC dataset at frequencies of 3.4% and 0.1%, for CLDN18-ARHGAP26 and CTNND1-ARHGAP26 , respectively. Fig. 3 Effect of fusions on the aggregation and proliferation of DGC cells ( a ) Slow aggregation assays of mouse DGC cells that stably expressed CLDN18-ARHGAP26 . Top panels, representative photographs (scale bar = 0.5 mm); Middle panels, cell aggregate diameter of DGC cells that stably expressed CLDN18-ARHGAP26 relative to cells expressing an empty vector. Average values for at least three independent experiments. Error bars, mean ± SEM. ( b ) Slow aggregation assays of mouse DGC cells that stably expressed Anxa2-Myo9a . Top panels, representative photographs (scale bar = 0.5 mm); Middle panels, cell aggregate diameter of DGC cells that stably expressed Anxa2-Myo9a relative to cells expressing an empty vector. Average values for at least three independent experiments. Error bars, mean ± SEM. # P < 0.05, * P < 0.01, **P < 0.001, *** P < 0.0001, paired t -test Full size image Another recurrent in-frame fusion, ANXA2-MYO9A , was identified in one early-onset and one late-onset case of DGC (Supplementary Figs. 5a and 5c ). Our study is the first to report this gene fusion in human cancer tissue samples. In both of the DGCs harboring the ANXA2-MYO9A fusion, ANXA2 exons 1‒4 (amino acids 1‒99) were fused in-frame to MYO9A exons 33‒42 (amino acids 1,994‒2,548) in the same orientation. Importantly, MYO9A exons 33‒42 included a RhoGAP domain. The ectopic expression of ANXA2-MYO9A in 293FT cells significantly suppressed Rho GTPase relative to the ectopic expression of an empty vector (Fig. 2d and Supplementary Fig. 4 ). These results suggest the biological relevance of the RhoGAP domain in the pathogenesis of this fusion. The early-onset DGC containing the ANXA2-MYO9A fusion had the highest MYO9A expression within the discovery set (Fig. 2e ). WGS data of this tumor revealed that g.chr15: 60,656,550 ( ANXA2 intron 4) was aberrantly fused to g.chr15: 72,157,966 ( MYO9A intron 32; Supplementary Table 9 ), which was confirmed by PCR sequencing analysis of genomic DNA (Fig. 2f ). Such rearrangement was not observed in adjacent normal tissue from the tumor sample, suggesting a somatic alteration (Supplementary Fig. 5b ). The tumors expressing the ANXA2-MYO9A fusion, an early-onset DGC and a late-onset DGC, demonstrated the stronger cytoplasmic and membranous MYO9A immunostaining than tumors without (P = 0.013, Cochran-Mantel-Haenszel; Fig. 2g and Supplementary Table 10 ). Thus, the three recurrent fusions each contained a RhoGAP domain in their 3’ partner genes. Proteins containing a RhoGAP domain usually function to inactivate RHO family small GTPases [23] . Notably, our mutation analyses revealed that CDH1 mutations, as well as RHOA mutations, were mutually exclusive with expression of the recurrent fusions. The three recurrent in-frame fusions were present in 17 of 384 patients with DGC, yet none of these 17 tumors contained CDH1 mutations. CDH1 mutations were present in 31.1% (66 of 212) of sequenced tumors without these fusions (P = 0.006, chi-square). In addition, no RHOA mutations were found among these 17 tumors, whereas 15.1% (32 of 212) of sequenced tumors without these fusions (P = 0.08, chi-square) had RHOA mutations, demonstrating a trend for mutual exclusivity. As with CLDN18-ARHGAP26 , the ectopic expression of Anxa2-Myo9a impaired the aggregation of mouse DGC cells ( Pdx1-cre ; Smad4 F/F ; Trp53 F/F ; Cdh1 F/+ cells, NCC-S1 cells, and NCC-S1M cells; P < 0.001, t -test; Fig. 3b and Supplementary Fig. 6 ). These data collectively suggest that RhoGAP domain-containing fusions may overlap with and RHOA [15] and CDH1 mutations in functional effect (Supplementary Fig. 7 ), and may underlie the poorly cohesive growth pattern of a subset of DGCs that are wild-type for RHOA and CDH1 . Clinicopathological correlates of RhoGAP domain fusions Among the 17 RhoGAP domain fusion-containing DGCs, only one tumor had the MSI and none were EBV-positive. The frequency of fusions did not vary with primary tumor location or gender (Fig. 4a ). While gastric cancer TCGA project reported that the CLDN18-ARHGAP26 fusion is enriched in the GS subgroup [3] , we found no difference in the distribution of TCGA molecular subgroup classifications between fusion-positive and fusion-negative DGCs within a larger sample set of DGCs (P = 0.7, chi-square; Fig. 4a ). Fig. 4 Clinical implications of RhoGAP domain-containing fusions in the expanded dataset (n = 384) ( a ) Clinicopathological characteristics (gender and primary tumor location) and TCGA subgroups in patients with (upper row) and without (lower row) RhoGAP domain-containing fusions. ( b ) Kaplan-Meier curves for the overall survival of patients with DGCs expressing three recurrent RhoGAP domain-containing fusions (n = 17) and those without (n = 367). ( c ) Kaplan-Meier curves for the overall survival of patients with DGCs expressing the CLDN18-ARHGAP26 fusion (n = 13) and those without (n = 371) Full size image Patients with RhoGAP domain fusion-containing DGCs (n = 17) had a significantly worse prognosis than those without such fusions (n = 367). The median survival was 29.1 [95% CI, 5.7‒not reached] and 94.6 [95% CI, 62.0‒not reached] months, respectively (P = 0.011, log-rank; Fig. 4b ; HR, 2.8 [95% CI, 1.5‒5.3]). Patients with these fusions tended to have more frequent distant metastasis at the time of diagnosis than those without, at 47.2% and 30.5%, respectively. However, this difference was not statistically significant (P = 0.15, chi-square; Fig. 4a ). Examining only patients with the CLDN18-ARHGAP26 fusion (n = 13) revealed a similarly poor prognosis as compared to patients without CLDN18-ARHGAP26 (Fig. 4c ). Specifically, patients with the CLDN18-ARHGAP26 fusion had a median survival of 26.9 months relative to 94.6 months for those without this fusion (n = 371; P = 0.001, log-rank; Fig. 4c ; HR, 2.2 [95% CI, 1.2‒4.1]). The prognostic impact of the CLDN18-ARHGAP26 fusion was comparable to that of the CDH1 mutation, which is a poor prognostic factor in early-onset DGC [15] (Supplementary Fig. 8 and Supplementary Tables 11 and 12 ). These results highlight the clinical relevance of RhoGAP-containing fusions, especially the CLDN18-ARHGAP26 fusion, in DGC. To gain functional insights into the poor prognostic role of CLDN18-ARHGAP26 in gastric cancer, we stably expressed CLDN18-ARHGAP26 in mouse gastric cancer cells. Phosphoproteome profiling analysis revealed that Regulation of actin cytoskeleton KEGG pathway phosphoproteins [24] , [25] , [26] , [27] , such as Actin-related protein 2, Actin-related protein 2/3 complex subunit 1B, and Profilin-1, were upregulated by CLDN18-ARHGAP26 (Supplementary Fig. 9 and Supplementary Table 13 ). Although mouse gastric cancer cells stably expressing CLDN18-ARHGAP26 did not significantly differ from empty vector-expressing cells in proliferation, epithelial-mesenchymal transition, tumorigenicity, and sphere-forming capacity (Supplementary Figs. 10 ‒ 14 ), migration ability was significantly enhanced following CLDN18-ARHGAP26 overexpression (Fig. 5a and Supplementary Fig. 15a ; P < 0.001, Wilcoxon signed rank test). To validate this finding, we evaluated the effect of CLDN18-ARHGAP26 overexpression on the migration ability of human gastric cancer cells. As in mouse gastric cancer cells, human gastric cancer cells (NUGC4, SNU-719, and SNU-638) stably expressing CLDN18-ARHGAP26 demonstrated a higher degree of migration ability than those expressing an empty vector (Fig. 5b and Supplementary Figs. 15b and 16 ; P < 0.001, Wilcoxon signed rank test). Ectopic expression of CLDN18-ARHGAP26 also enhanced the invasion capacity of these human gastric cancer cells (Fig. 5c ; P < 0.001, Wilcoxon signed rank test). These functional data suggest that CLDN18-ARHGAP26 confers the metastatic phenotype on gastric cancer by enhancing migration and invasion capacities. Fig. 5 Functional effects of CLDN18-ARHGAP26 overexpression ( a ) Top, Trans-well migration assay. Mouse gastric cancer cells stably expressing CLDN18-ARHGAP26 demonstrated significantly enhanced migration ability compared with those expressing an empty vector (P < 0.001, Wilcoxon signed rank), and this effect was prominent in NCC-S1M and Pdx1-cre;Smad4 F/F ; Trp53 F/F ; Cdh1 F/+ cells. Vertical axis denotes the normalized number of migrated cells per field. Average values of 4 independent experiments; Bottom, RT-PCR for CLDN18-ARHGAP26 ( b ) Top, Migration assay of human gastric cancer cells following the ectopic expression of CLDN18-ARHGAP26 . Human gastric cancer cells stably CLDN18-ARHGAP26 demonstrated significantly enhanced migration capacity compared with those expressing an empty vector (P < 0.001, Wilcoxon signed rank). Vertical axis denotes the normalized number of migrated cells per field. Average values of 3 independent experiments; Bottom, RT-PCR for CLDN18-ARHGAP26 . ( c ) Left, Invasion assay. Human gastric cancer cells stably expressing CLDN18-ARHGAP26 demonstrated significantly enhanced invasion capacity compared with those expressing an empty vector (P < 0.001, Wilcoxon signed rank). Vertical axis denotes the normalized number of migrated cells per field. Average values of three independent experiments. Right, Representative photographs of the invasion assay (200 × , scale bar = 0.2 mm). 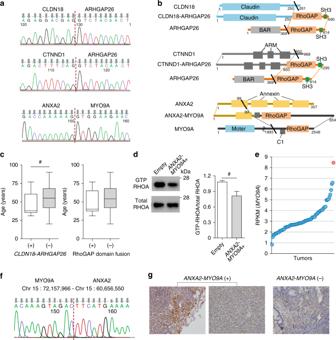Red arrows, gastric cancer cells. Error bars, mean ± SEM. # P < 0.05, *P < 0.01, **P < 0.001, ***P < 0.0001 Full size image TACC2-PPAPDC1A identified as another recurrent fusion To extend our initial findings from RNA sequencing and RT-PCR analyses, we then conducted targeted RNA sequencing analyses for all exons from the 25 in-frame gene fusions first identified by RNA sequencing analysis of the discovery set. The expanded dataset DGCs without available RNA sequencing data (n = 225) were subjected to targeted RNA sequencing analyses, with the mean sequencing coverage of 56.1-fold. Fig. 2 Schematic representation of three recurrent RhoGAP domain-containing fusions (a) Chromatogram for the RT-PCR sequencing data. Dotted red lines, mRNA breakpoints. (b) Top panel, theCLDN18-ARHGAP26fusion. Middle panel, theCTNND1-ARHGAP26fusion was composed of the Armadillo (Arm) family domain ofCTNND1that is involved in cell-cell adhesion and signal transduction and RhoGAP and SH3 domains ofARHGAP26. Bottom panel, theANXA2-MYO9Afusion was composed of 99 amino acids in the N-terminal portion ofANXA2and the protein kinase C conserved region 1 (C1) and RhoGAP domain ofMYO9A. (c) Left panel, Age at the time of diagnosis was significantly lower in patients with theCLDN18-ARHGAP26fusion (n = 13; left) than in those without (n = 371; right) (P = 0.042, Wilcoxon). Right panel, Age tended to be lower in patients with RhoGAP domain-containing fusions (n = 17; left) than those without (n = 367; right) (P = 0.10, Wilcoxon). Box plots display 5%, 25%, median, 75%, and 95%. (d) RhoTekin assay in 293FT cells following the ectopic expression ofAnxa2-Myo9afusion. Relative value of GTP-RHOA to total RHOA as measured by a densitometry in three independent experiments. Error bars, mean ± SEM. (e) RPKM values forMYO9Ain 80 early-onset DGCs (dots) in a discovery dataset. Each circle represents each tumor. Blue circle, a tumor expressing theANXA2-MYO9Afusion. (f) PCR sequencing chromatogram for genomic DNA isolated from a tumor expressing theANXA2-MYO9Afusion. Dotted line, chromosomal breakpoint. (g) MYO9A immunohistochemistry images were taken at 200 × . Left, Two DGCs expressing theANXA2-MYO9Afusion. Right, Representative photographs for a randomly-selected DGC without theANXA2-MYO9Afusion (P = 0.013;ANXA2-MYO9A-positive tumors vs.ANXA2-MYO9A-negative tumors; Cochran-Mantel-Haenszel).#P < 0.05, *P < 0.01, **P < 0.001, ***P < 0.0001, Error bar, mean ± SEM We identified additional novel gene fusions harboring mRNA breakpoints that were different from those initially discovered (Table 2 ). In the 225 DGCs, targeted RNA sequencing analyses revealed three additional CLDN18-ARHGAP26 fusion events, two of which had mRNA breakpoints distinct from breakpoints identified by RNA sequencing analysis of the discovery set. More importantly, targeted RNA sequencing identified two additional TACC2-PPAPDC1A fusion events with an mRNA breakpoint different from the breakpoint initially discovered (Fig. 6a ). Thus, we identified a novel recurrent in-frame fusion present in 1% of tumors (3 of 305) sequenced by either RNA sequencing or targeted RNA sequencing analyses. Our study is the first to report TACC2-PPAPDC1A as a recurrent fusion gene in human cancer tissue samples, although PVT1-PPAPDC1A has been reported to be present in a gastric cancer cell line [20] . In the early-onset, discovery set DGC harboring TACC2-PPAPDC1A , TACC2 exons 1‒6 (amino acids 1‒1899) were fused in-frame to PPAPDC1A exons 2‒7 (amino acids 20‒271) in the same orientation. In the other two DGCs with this fusion, TACC2 exons 1‒3 (amino acids 1‒48) were also fused in-frame to PPAPDC1A exons 2‒7 (amino acids 20‒271) in the same orientation. No TACC2-PPAPDC1A transcripts were present in normal adjacent tissue of the three tumors, suggesting their somatic nature. Table 2 In-frame gene fusions additionally identified by targeted RNA sequencing analysis Full size table Fig. 6 The PPAPDC1A in-frame fusions identified by targeted RNA sequencing ( a ) Schematic representation of the PPAPDC1A fusions. Top and middle panels, TACC2-PPAPDC1A fusions; Bottom panel, ARIH1-PPAPDC1A . CC, Coiled-coil domain; PAP2, PAP2 domain; ZF, Zinc finger domain. ( b ) Left, PPAPDC1A RPKM values for the 80 discovery set DGCs. Each circle represents each tumor. Sample ordering according to the PPAPDC1A RPKM. Magenta circle, early-onset DGC expressing TACC2- PPAPDC1A . Right, PPAPDC1A RPKM values for the discovery set DGCs with and without 10q26.1 gene amplification. Turquoise circle, early-onset DGC expressing TACC2- PPAPDC1A . Box plots display 5%, 25%, median, 75%, and 95%. ( c ) Lipidomic profiling data for DGCs with or without TACC2-PPAPDC1A . The sum of the mass spectral peak area ratio between phosphatidic acid (PA, the substrate of PPAPDC1A) and diacylglycerol (DG, the product of PPAPDC1A) was significantly lower in an early-onset DGC expressing TACC2-PPAPDC1A in the discovery set than in randomly-selected eight DGCs without the fusion (P = 0.01, one-sample rank sum test). Vertical axis denotes the sum of mass spectral peak area ratio between PA and the corresponding DG for each PA-DG pair. Each circle represents each tumor. Magenta circle, early-onset DGC expressing TACC2- PPAPDC1A . # P value for an one-sample rank sum test. Box plots display 5%, 25%, median, 75%, and 95% Full size image RNA sequencing analysis revealed that the early-onset DGC containing TACC2-PPAPDC1A displayed the highest PPAPDC1A expression and expressed higher levels of PPAPDC1A mRNA than tumors with 10q26.1 gene amplification (Fig. 6b ). Tissue distribution of PPAPDC1A ( DPPL2 ) mRNA expression is restricted mainly to the brain, kidney and testes, with no endogenous PPAPDC1A expression in the stomach [28] . In DGCs carrying TACC2-PPAPDC1A, PPAPDC1A overexpression was presumably driven by the TACC2 promoter, as a result of the in-frame fusion event. Mass spectrometry-based, lipidomic profiling analyses [29] suggested relatively high phospholipid phosphatase activity in the early-onset DGC expressing TACC2-PPAPDC1A (P = 0.01, one-sample rank sum test; Fig. 6c and Supplementary Fig. 17 ). This finding suggests that the possible functional relevance of the TACC2-PPAPDC1A , although further biochemical validation is needed. All three patients with TACC2-PPAPDC1A gene fusions were male, and their median age (67 years) did not differ from the 302 sequenced dataset DGCs without the fusion (P = 0.51 , t -test). One of the three tumors belonged to the CIN subgroup, while the other two tumors were in the GS subgroup. Thus, the distribution of TCGA subgroup and primary tumor location was not different according to TACC2-PPAPDC1A status. Patients with TACC2-PPAPDC1A tended to exhibit more frequent distant metastasis at the time of diagnosis (66.6%) than those without (24.5%; P = 0.15, Fisher’s exact test; Fig. 7a ). Consistently, patients with DGCs expressing TACC2-PPAPDC1A had a significantly worse prognosis than those without such fusions. The median survival time for those with TACC2-PPAPDC1A was 3.5 months [95% CI, 0.5‒not reached], while a median survival time was not reached among those without [95% CI, 61.8‒not reached; P < 0.0001, log-rank; HR, 8.6 [95% CI, 2.7‒27.3]; Fig. 7b ). Two of the three tumors harbored gene amplifications in the 10q26.1 locus, whereas the third tumor contained CDH1 mutations. We observed, however, that the prognostic impact of TACC2-PPAPDC1A was independent of 10q26.1 amplification and CDH1 mutations (adjusted HR, 7.1 [95% CI, 2.1‒23.6]; Supplementary Table 14 ). Fig. 7 Clinical implications of the TACC2-PPAPDC1A fusion in the sequenced dataset (n = 305) ( a ) Stage at the time of diagnosis and TCGA subgroups in patients with or without TACC2-PPAPDC1A . TCGA subgroup was determined only in DGCs with available SNP6.0 data. ( b ) Kaplan-Meier curves for the overall survival of three patients with DGCs expressing TACC2-PPAPDC1A and those without (n = 302). Their median survival times were 3.5 months and not reached, respectively (P < 0.0001, log-rank). ( c ) Kaplan-Meier curves for the overall survival of four patients with DGCs expressing PPAPDC1A fusions and those without (n = 301). Their median survival times were 12.1 months and not reached, respectively (P < 0.0001, log-rank; HR, 6.6 [95% CI, 2.4‒18.1]). ( d ) Kaplan-Meier curves for the overall survival of 23 patients with the PPAPDC1A or RhoGAP domain-containing fusions and those without (n = 282). Their median survival times were 22.8 months [95% CI, 5.7‒33.0] and not reached, respectively (P < 0.0001, log-rank; HR, 3.4 [95% CI, 2.0‒5.7]) Full size image In addition to TACC2 , another in-frame fusion event with PPAPDC1A was observed with ARIH1 as the 5’ partner gene. In this DGC, ARIH1 exons 1‒2 (amino acids 1‒147) at chromosome 15 were fused in-frame to PPAPDC1A exons 2‒7 (amino acids 20‒271) at chromosome 10 (Fig. 6a ). Thus, all four PPAPDC1A fusion events included the PAP2 (type 2 phosphatidic acid phosphatase) domain as the 3’ partner gene, and no PPAPDC1A fusion transcripts were present in normal adjacent tissue. When all four PPAPDC1A fusions were considered, PPAPDC1A continued to be a strong prognostic indicator, independent from 10q26.1 gene amplification (adjusted HR, 7.8 [95% CI, 2.3‒25.8]; Fig. 7c ). Actionable FGFR2-TACC2 identified by targeted RNA sequencing Interestingly, 5 of 18 in-frame fusions identified by our targeted RNA sequencing were located at the chromosome locus 10q26.1 (Table 2 ; P = 0.002, chi-square). One such novel in-frame fusion involving this locus was FGFR2-TACC2 . Given that FGFR1-TACC1 and FGFR3-TACC3 play oncogenic roles in several solid tumors [30] , this novel fusion might contribute to DGC carcinogenesis through activation of the FGFR2 kinase mediated by the coiled-coil domain of TACC2. Notably, FGFR2-TACC2 is clinically-actionable, similar to EML4-ALK as described above. Thus, our comprehensive in-frame fusion screen determined that 0.7% (2 of 305) of the sequenced dataset DGCs harbor clinically-actionable fusions. Table 2 summarizes in-frame gene fusions additionally identified by targeted RNA sequencing analysis. All fusions, except CLDN18-ARHGAP26 , represent novel discoveries related to DGCs. Included in this list was VMP1-RPS6KB1 , which was previously reported in breast cancer and esophageal adenocarcinomas [21] , [31] , but not in gastric cancer. 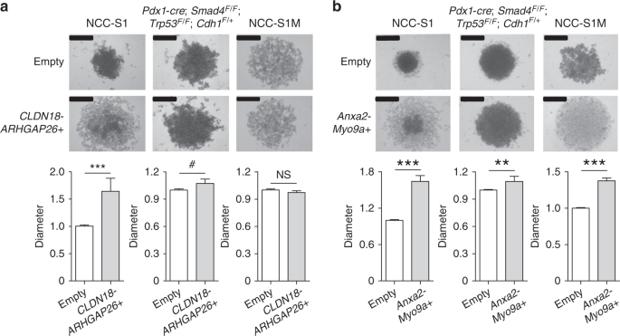Recurrent fusions defined the subgroup with worst prognosis Our comprehensive in-frame fusion screen using the largest-ever set of DGCs identified the TACC2-PPAPDC1A and RhoGAP domain-containing in-frame fusions as recurrent somatic alterations. Presence of one of these recurrent in-frame fusions ( TACC2-PPAPDC1A , CLDN18-ARHGAP26 , CTNND1-ARHGAP26 , or ANXA2-MYO9A ) was associated with very poor prognosis. The median survival time for those with recurrent fusions was 22.8 months [95% CI, 5.0‒33.0], while a median survival time was not reached among those without recurrent fusions (P < 0.0001, log-rank; HR, 3.5 [95% CI, 2.0‒6.0]). Univariate survival analyses indicated that chromosomal instability (CIN), which was determined by parallel SNP6.0 array analyses [15] , and CDH1 mutation were significant prognostic genomic alterations in our DGCs, consistent with our previous report [15] (HRs, 2.3 [95% CI, 1.3‒3.9] and 1.8 [95% CI, 1.1‒3.0], respectively), whereas TP53 mutations were not (P = 0.80, log rank). Fig. 3 Effect of fusions on the aggregation and proliferation of DGC cells (a) Slow aggregation assays of mouse DGC cells that stably expressedCLDN18-ARHGAP26. Top panels, representative photographs (scale bar = 0.5 mm); Middle panels, cell aggregate diameter of DGC cells that stably expressedCLDN18-ARHGAP26relative to cells expressing an empty vector. Average values for at least three independent experiments. Error bars, mean ± SEM. (b) Slow aggregation assays of mouse DGC cells that stably expressedAnxa2-Myo9a. Top panels, representative photographs (scale bar = 0.5 mm); Middle panels, cell aggregate diameter of DGC cells that stably expressedAnxa2-Myo9arelative to cells expressing an empty vector. Average values for at least three independent experiments. Error bars, mean ± SEM.#P < 0.05,*P < 0.01, **P < 0.001,***P < 0.0001, pairedt-test According to Cox regression analysis, the prognostic impact of recurrent in-frame fusions (adjusted HR, 4.3 [95% CI, 2.1‒8.4]) was independent of the chromosomal instability and the CDH1 mutation (Table 3 ). Overall, the PPAPDC1A and RhoGAP domain-containing in-frame fusions were present in 7.5% (23 of 305) of the sequenced dataset DGCs, but not in adjacent normal tissue. These fusions clearly defined the subset of aggressive DGCs (HR, 3.4 [95% CI, 2.0‒5.7]; Fig. 7d ), and their prognostic impact was higher than, and independent of, the chromosomal instability and the CDH1 mutation (Table 3 ). Table 3 Cox regression survival analysis of 173 DGCs with available SNP6.0 array and DNA sequencing data Full size table In this study, we investigated the biological and clinical implications of fusion genes in early-onset DGCs. According to RNA sequencing and RT-PCR analyses, three in-frame fusions were recurrent. All these three contained a RhoGAP domain [23] in their 3’ region (Fig. 2b ), suggesting that this domain may have biological relevance to the pathogenesis of fusions in DGC. The RHO family is comprised of small G proteins that are inactivated by GTPase-activating proteins by stimulating the intrinsic GTPase activity of small G proteins. The C-terminal end of ARHGAP26 and the effector region of MYO9A were conserved in fusion genes, suggesting that the Rho family GTPase pathway is a primary target of recurrent in-frame fusion transcripts in DGC [3] . This study is the first to demonstrate that the three RhoGAP domain-containing fusions were mutually exclusive with CDH1 mutations in DGC. Previous reports have suggested that the CLDN18-ARHGAP26 fusion is mutually exclusive with RHOA mutations [3] , which corresponds with observations in the current study. Mutations in CDH1 and RHOA impair cell adhesion in a process characteristic of DGC pathogenesis. Given that these fusions were mutually exclusive with CDH1 and RHOA mutations but impaired cell aggregations in a manner similar to such mutations, RhoGAP domain-containing fusions may play a role in the development of the poorly cohesive growth pattern characteristic of DGC. Interestingly, the CLDN18-ARHGAP26 fusion was significantly more common in younger patients than in older patients, as with the ALK or RET fusions in lung adenocarcinomas [10] , [11] . A majority of gastric cancers in young patients exhibits diffuse type histology, and RhoGAP domain-containing recurrent fusions were more prevalent in the diffuse type than in the intestinal type (P = 0.03, chi-square; Supplementary Table 15 ). We also observed a trend for the relatively high prevalence of the CLDN18-ARHGAP26 fusion among H. pylori -positive DGCs. The association between H. pylori and chromosomal translocation has not been reported in gastric adenocarcinomas, unlike in MALT lymphomas. Further studies are warranted to validate this interesting finding. Another novel recurrent fusion, ANXA2-MYO9A , resulted from an intrachromosomal rearrangement and led to the overexpression of its 3’ partner gene, MYO9A . Myosin 9 A (Myr7) contains the RhoGAP domain and is an actin-dependent motor protein of the unconventional myosin IX class. The RhoGAP domain enables class IX myosins to inactivate small GTPases of the Rho family [32] . Specifically, Myr7 inactivates Rho by stimulating its GTPase activity in neurons [23] , [33] . MYO9A is expressed in several tissues and is enriched in the brain and testes [33] , [34] . Myo9a knockout mice develop hydrocephalus and kidney dysfunction, which highlights the importance of MYO9A in epithelial cell morphology and differentiation [35] , [36] . ANXA2 encodes Annexin A2, a calcium-regulated membrane-binding protein [37] . MYO9A was overexpressed in the tumor containing the ANXA2-MYO9A fusion, which supports transcriptional activation as the oncogenic mechanism for this gene fusion. Our cell aggregation data regarding ectopic expression of CLDN18-ARHGAP26 are consistent with Yao et al.’s data studying the effect of this same fusion in HGC27 cells [9] . Yao et al. suggested that CLDN18-ARHGAP26 fusion compromises the role of CLDN18 in epithelial barrier promotion and directly affects the intactness of the paracellular barrier [9] . Given our RNA sequencing and RT-PCR data that all recurrent in-frame fusions contain RhoGAP domain, functional alteration of ARHGAP26 might possibly be more important than that of impaired CLDN18 function in the oncogenic mechanism of CLDN18-ARHGAP26 fusion. Given that cell migration/invasion activities are regulated by complex crosstalk between RHO GTPases [38] , [39] , [40] , further biochemical studies are warranted to explore how CLDN18-ARHGAP26 affect the migration/invasion activities of gastric cancer cells. Our targeted RNA sequencing analysis [41] was the first to reveal that DGC’s in-frame fusion events frequently involved the chromosomal fragile site at 10q26.1 that harbors TACC2, FGFR2 , and PPAPDC1A , in addition to RhoGAP domain-containing genes. This result may be consistent with our previously reported genomic data, which identified the chromosomal locus 10q26.1 as the most recurrent focal gene amplification in Korean DGCs [15] . Although the 10q26.1-amplified gastric cancer cell line SNU16 expresses PVT1-PPAPDC1A [20] , PPAPDC1A fusion events have not been reported recurrent in human gastric cancers. While our analysis was limited by the relatively small number of PPAPDC1A fusion events in our dataset, the prognostic impact of PPAPDC1A fusions was higher than, and independent of, that of 10q26.1 gene amplification. PPAPDC1A encodes a phospholipid phosphatase that converts phosphatidic acids to diacylglycerols [42] , and our lipidomic profiling data suggested the biochemical relevance of TACC2-PPAPDC1A mRNA expression. While we cannot rule out a possibility that PPAPDC1A fusions may just represent the genomic instability of DGCs, our findings warrant further functional studies that evaluate potentiality of PPAPDC1A fusions’ use as therapeutic targets such as neoantigens in personalized immunotherapy. Compared to intestinal-type gastric cancer, DGC has not been fully investigated for prognostic factors despite its significant worldwide disease burden [1] , [2] . We previously reported that CIN, followed by CDH1 alteration, is the most adverse prognostic factor in early-onset DGCs [15] . Our current, comprehensive study systematically explored recurrent in-frame somatic fusions, excluding less clinically relevant fusion events such as read-through transcripts. In addition, rigorous RT-PCR analyses of tumors and adjacent normal tissue validated the somatic nature of novel in-frame fusions. Similar genomic studies have not yet been conducted on adequately-sized DGC sets with long-term follow up. Thus, here we present the first genomic study that clearly demonstrates the prognostic impact of novel recurrent PPAPDC1A and RhoGAP domain-containing fusions, which was more prominent than those of the chromosomal instability and CDH1 mutations. These fusions partially overlapped with CIN tumors, but their prognostic impact was independent of that of CIN. In summary, our findings suggest possible roles that RhoGAP and PAP2 domains play in cancer progression and provide novel genomic insights guiding future strategies for managing DGCs. Patients This study was approved by the National Cancer Center Institutional Review Board (IRB; NCCNCS-120581), and all patients signed IRB-approved consent forms. RNA sequencing analyses were performed in 80 resected tumors and 65 normal tissue adjacent to the 80 tumors that had RNA sequencing data. These tissue samples were collected from patients with early-onset ( ≤ 45 years) DGCs (discovery dataset). For RT-PCR analysis of gene fusions, the dataset was expanded to 384 biopsy and surgical DGC samples (Supplementary Table 1 ). To estimate the sample size required for an expanded dataset, we hypothesized that recurrent in-frame fusions are present in 15% of tumors and adversely affect prognosis by a hazard ratio of 2. At two-tailed α and β errors of 0.05 and 0.2, respectively, 128 events were estimated to be required to evaluate the effect of fusions on survival [43] . We assumed that about one third of patients with advanced stage gastric cancers die during 3-year follow-up [44] . For 128 events, therefore, 384 tumors were estimated to be required as an expanded dataset. RNA sequencing and the identification of novel fusions Transcriptome libraries were prepared using poly(A) + RNA isolated from 1–2 μg of total RNA from frozen macrodissected tumors in a discovery dataset and TruSeq mRNA Kit (Illumina, San Diego, CA). Paired-end libraries were sequenced using an Illumina HiSeq 2000 instrument (2 × 100 nucleotide read length). RNA-seq Data Analysis (PRADA) [45] , [46] was used for fusion discovery. Using the preprocess module of PRADA, we aligned RNA sequencing reads on human reference genome hg19/GRCh37 and human transcripts of Ensembl build 64. We discovered gene fusion candidates using the fusion module, and selected in-frame fusion candidates using the prada-frame utility. In parallel, deFuse [47] , FusionMap [48] , and TopHat-Fusion [49] were additionally used to predict candidate fusion breakpoints (Supplementary Fig. 19 ). To remove false-positive breakpoints resulting from these algorithms, we reconstructed candidate regions containing putative breakpoints using Trans-ABySS [50] , [51] (v1.4.4). Trans-ABySS performed a de novo assembly on candidate regions containing putative breakpoints that were identified by deFuse, FusionMap and TopHat-Fusion. We then performed RT-PCR sequencing analyses to validate the expression of candidate fusions that were in-frame and contained partner genes of importance based on the data in the literature (Supplementary Fig. 19 and Supplementary Table 5 ). RT-PCR analysis of mRNA breakpoints and mutation analyses Total RNA samples from the expanded dataset were subjected to RT-PCR analyses of 25 validated in-frame fusions. Synthesized cDNA was PCR-amplified for 35 cycles. Mutations in CDH1, RHOA and TP53 were identified by targeted DNA sequencing analyses [15] . Cell lines and lentiviral vectors NCC-S1 and NCC-S1M cell lines were established by our group from a diffuse-type gastric adenocarcinoma formed in a Villin-cre ; Smad4 F/F ; Trp53 F/F ; Cdh1 F/+ mouse [52] , [53] . Pdx1-cre;Smad4 F/F ; Trp53 F/F ; Cdh1 F/+ cells were primary cultured by our group from a diffuse-type gastric adenocarcinoma formed in a Pdx1-cre; Smad4 F/F ; Trp53 F/F ; Cdh1 F/+ mouse [52] , [53] . To generate the Anxa2-Myo9a lentiviral expression vector, mouse genomic DNA sequences that were homologous to human ANXA2-MYO9A ( Anxa2 coding sequence 1‒300 and Myo9a coding sequence 6,694‒7,896) were synthesized and subcloned using a pCDH-CAG-MSC-EF1-Neomycin vector. For the CLDN18-ARHGAP26 lentiviral vector, CLDN18 coding sequence 1‒750 and ARHGAP26 coding sequence 1,108‒2,280 were ligated and cloned using a pCDH-CAG-MSC-EF1-Puromycin vector. Targeted RNA sequencing analysis Of the 304 expanded dataset DGCs without available RNA sequencing data, 225 tumors (74%) were subjected to a hybrid capture-based, custom targeted RNA sequencing analysis [38] . These 225 DGCs were combined with the 80 DGCs with available RNA sequencing data and this combined dataset (sequenced dataset (n = 305)) was used to determine frequencies of PPAPDC1A fusions (Supplementary Table 2 ). Hybrid capture probes were designed to cover all the exons of 25 in-frame fusions listed in Table 1 . SureSelect RNA Direct (Agilent Technologies, Santa Clara, CA) was used for library construction. Gene fusions were identified using deFuse [47] with default parameters. In-frame fusion transcripts with > 3 spanning reads were identified as fusion candidates, and were confirmed by RT-PCR sequencing analyses (Table 2 ). Code availability The source code of a program to predict if an RNA sequence is in frame is available from the corresponding author on reasonable request.